Genome-scale proteome quantification by DEEP SEQ mass spectrometry Advances in chemistry and massively parallel detection underlie DNA-sequencing platforms that are poised for application in personalized medicine. In stark contrast, systematic generation of protein-level data lags well behind genomics in virtually every aspect: depth of coverage, throughput, ease of sample preparation and experimental time. Here, to bridge this gap, we develop an approach based on simple detergent lysis and single-enzyme digest, extreme, orthogonal separation of peptides and true nanoflow liquid chromatography-tandem mass spectrometry that provides high peak capacity and ionization efficiency. This automated, deep efficient peptide sequencing and quantification mass spectrometry platform provides genome-scale proteome coverage equivalent to RNA-seq ribosomal profiling and accurate quantification for multiplexed isotope labels. In a model of the embryonic to epiblast transition in murine stem cells, we unambiguously quantify 11,352 gene products that span 70% of Swiss-Prot and capture protein regulation across the full detectable range of high-throughput gene expression and protein translation. The field of DNA and RNA sequencing has progressed at a remarkable rate since release of the initial human genome draft sequences [1] , [2] . Genotype–phenotype association studies continue to elucidate large genomic regions that are amplified, deleted or otherwise altered in the context of human disease, although identification of specific causal gene elements has proven to be a significant challenge [3] . Despite these and other successes [4] , primary DNA sequence data does not capture downstream regulatory information for protein translation, degradation and post-translational modification status [5] , [6] , [7] . These data are critical components of studies designed to quantitatively monitor biological response to perturbation or build predictive models of cellular physiology [8] . As a result, there remains a clear and unmet need for methodologies that can provide systematic and scalable sequence characterization of proteins as an important functional complement to DNA and RNA data. The wide dynamic range of protein expression and vast array of post-translational modifications, coupled with the lack of an analyte amplification strategy analogous to PCR, presents tremendous challenges for genome-wide protein characterization, particularly for signal transduction and other key regulatory factors that are often present in low abundance. As a result, the majority of shotgun sequencing approaches frequently rely on low-throughput pre-fractionation (for example, before liquid chromatography-tandem mass spectrometry (LC-MS/MS) analysis) of sub-cellular compartments or intact proteins to improve dynamic range. Although these techniques are subject to continued improvements, they have not yet achieved genome-scale protein identification and quantification. Moreover, in many cases the labour-intensive nature of pre-fractionation protocols hinders widespread adoption and standardization. In this work, we forgo cellular- or protein-level pre-fractionation altogether and instead rely on direct detergent-based protein solubilization, followed by single-enzyme trypsin digest and extensive, fully automated temporal separation of peptides through multiple physicochemically orthogonal stages: high-pH reversed phase (RP) and strong anion exchange (SAX) dimensions coupled in series and directly with a narrow-bore, extended-length (25 μm × 100 cm) low-pH RP analytical column operated in a true nanoflow regime. The latter chromatographic stage provides high peak capacity separation in a third orthogonal dimension, along with increased electrospray ionization efficiency for improved detection. The figures of merit for these individual components combine to yield an automated DEep Efficient Peptide SEquencing and Quantification (DEEP SEQ) mass spectrometry platform that provides unprecedented separation capacity, rapid sequencing speed and quantification of proteins across the entire range of mammalian gene expression and protein translation. We utilized multiplexed stable isotope labels in the context of a model designed to profile early perturbations in the naive, self-renewing ground state of murine embryonic stem cells (mESCs) to quantify 211,535 unique peptide sequences that mapped unambiguously to 11,352 gene products. These results span ~70% of the highly curated Swiss-Prot database, capture a vast majority of known pluripotency factors and provide a depth and scale of proteome coverage commensurate with genome-wide analysis of protein translation by RNA-seq ribosomal profiling [9] . Peptide quantification by DEEP SEQ mass spectrometry Multiplexed isotope labels have emerged as an enabling technology to increase the throughput of quantitative proteomic studies and provide increased flexibility with respect to experimental variables (time course, dose response and so on) [10] . As these reagents have enjoyed wider use, it has become apparent that quantification accuracy degrades significantly as the complexity of target analyte mixtures increases. Simultaneous fragmentation of precursors that overlap in m/z leads to a compression of discrete peptide ratios towards the mean of all measured values [11] , [12] , [13] . We reasoned that the extreme temporal separation provided on our protein deep-sequencing platform would mitigate deleterious ratio compression effects. To explore this hypothesis, we created a mixed-species quantification model [12] , [13] in which the contaminant peptides were present at a mass ratio of ~6- and ~32-fold greater as compared with the target species, respectively ( Fig. 1a ). We acquired data at a depth of 20 DEEP SEQ fractions (Methods) with an LTQ-Orbitrap XL and used multiplierz [14] , [15] to compile and analyse extracted ion chromatograms for all detected peptides. We observed an average chromatographic peak width measured at half-height of 27.8 s ( Fig. 1b ), with over 97% of all detected peptides spanning no more than two adjacent fractions ( Fig. 1c ), yielding an empirical peak capacity [16] of ~1.3 E4. Importantly, projection of peptide sequence identifications as a function of first-dimension organic and second-dimension salt concentrations ( Fig. 1d ) revealed that peptides were distributed throughout the entire separation space, confirming that our platform provided orthogonal and extensive peptide separation in these experiments. We next plotted isobaric tags for relative and absolute quantitation (iTRAQ) ratios for species-specific peptides and compared these with ratios observed in a conventional, single-dimension LC-MS/MS analysis of the same sample mixture. The median ratio for the mixed-species channels (116:114) in the standard LC-MS/MS analysis was compressed by some 40% as compared with the single-species ratios (117:115); however, the equivalent analysis with DEEP SEQ mass spectrometry revealed a relative ratio compression of only 8% ( Fig. 1e and Supplementary Data 1 ). Inspection of individual peptide spectra ( Fig. 1f ) reveals the marked improvement in quantification data provided by our DEEP SEQ platform. 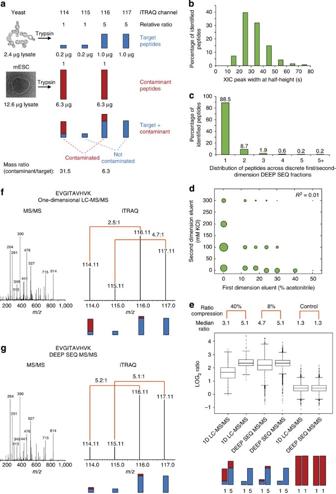Figure 1: DEEP SEQ mass spectrometry provides extreme separation and accurate quantification of iTRAQ-labelled peptides. (a) A mixed-species iTRAQ quantification model consisting of tryptic target peptides from yeast: 0.2 μg (iTRAQ 114), 0.2 μg (iTRAQ 115), 1.0 μg (iTRAQ 116) and 1.0 μg (iTRAQ 117), and contaminant peptides from mESCs: 6.3 μg (iTRAQ 114) and 6.3 μg (iTRAQ 116). Contaminant peptides are 6.3 × and 31.5 × more abundant in the iTRAQ 116 and 114 channels, respectively, as compared with the yeast target peptides. (b) Histogram of extracted ion chromatogram peak width for peptides identified in 20-fraction DEEP SEQ MS/MS analysis of mixed-species model. (c) Analysis of peptide-elution profiles demonstrates minimal fraction-to-fraction overlap, with ~97% of all identified peptides constrained within two adjacent first/second-dimension (high-pH RP/SAX) fractions. (d) The number of identified peptides represented as circles of proportional diameter and plotted as a function of first/second-dimension eluent concentration; low correlation coefficient for least-squares fit of these data (R2=0.01) suggests orthogonal fractionation of peptides across high-pH RP and strong anion-exchange dimensions. (e) Log2iTRAQ ratios of peptides identified in the mixed-species model displayed in box-plot format for conventional single-dimension LC-MS/MS and DEEP SEQ analyses. The data include 272 yeast-specific peptides and 1570 mouse-specific peptides in one-dimensional mode, along with 2,446 yeast-specific and 20,461 mouse-specific peptides, identified in the DEEP SEQ analysis. Boxes encompass the interquartile range with respective median values indicated with stripes; whiskers represent 1.5 × the interquartile range with outliers shown as open circles. Non-transformed, median ratios are listed at the top along with relative ratio compression for contaminated (116:114, blue+red) versus non-contaminated (117:115, blue) iTRAQ ratios. Analysis of mESC contaminant peptides alone (two right-most box plots) provides a positive control for iTRAQ ratios measured in conventional LC-MS/MS and DEEP SEQ analyses, respectively. (f,g) Representative MS/MS spectra for a tryptic peptide (EVGITAVHVK) acquired during (f) typical shotgun LC-MS/MS and (g) DEEP SEQ mass spectrometry analyses. Low-massm/zregion shows iTRAQ signals for each fragment ion spectrum along with measured ratios for contaminated (116:114, blue+red) and non-contaminated (117:115, blue) channels. Figure 1: DEEP SEQ mass spectrometry provides extreme separation and accurate quantification of iTRAQ-labelled peptides. ( a ) A mixed-species iTRAQ quantification model consisting of tryptic target peptides from yeast: 0.2 μg (iTRAQ 114), 0.2 μg (iTRAQ 115), 1.0 μg (iTRAQ 116) and 1.0 μg (iTRAQ 117), and contaminant peptides from mESCs: 6.3 μg (iTRAQ 114) and 6.3 μg (iTRAQ 116). Contaminant peptides are 6.3 × and 31.5 × more abundant in the iTRAQ 116 and 114 channels, respectively, as compared with the yeast target peptides. ( b ) Histogram of extracted ion chromatogram peak width for peptides identified in 20-fraction DEEP SEQ MS/MS analysis of mixed-species model. ( c ) Analysis of peptide-elution profiles demonstrates minimal fraction-to-fraction overlap, with ~97% of all identified peptides constrained within two adjacent first/second-dimension (high-pH RP/SAX) fractions. ( d ) The number of identified peptides represented as circles of proportional diameter and plotted as a function of first/second-dimension eluent concentration; low correlation coefficient for least-squares fit of these data ( R 2 =0.01) suggests orthogonal fractionation of peptides across high-pH RP and strong anion-exchange dimensions. ( e ) Log 2 iTRAQ ratios of peptides identified in the mixed-species model displayed in box-plot format for conventional single-dimension LC-MS/MS and DEEP SEQ analyses. The data include 272 yeast-specific peptides and 1570 mouse-specific peptides in one-dimensional mode, along with 2,446 yeast-specific and 20,461 mouse-specific peptides, identified in the DEEP SEQ analysis. Boxes encompass the interquartile range with respective median values indicated with stripes; whiskers represent 1.5 × the interquartile range with outliers shown as open circles. Non-transformed, median ratios are listed at the top along with relative ratio compression for contaminated (116:114, blue+red) versus non-contaminated (117:115, blue) iTRAQ ratios. Analysis of mESC contaminant peptides alone (two right-most box plots) provides a positive control for iTRAQ ratios measured in conventional LC-MS/MS and DEEP SEQ analyses, respectively. ( f , g ) Representative MS/MS spectra for a tryptic peptide (EVGITAVHVK) acquired during ( f ) typical shotgun LC-MS/MS and ( g ) DEEP SEQ mass spectrometry analyses. Low-mass m/z region shows iTRAQ signals for each fragment ion spectrum along with measured ratios for contaminated (116:114, blue+red) and non-contaminated (117:115, blue) channels. Full size image Genome-wide protein quantification comparable to ribo-seq To further explore the performance of our protein deep-sequencing platform, we sought to quantify changes in mESC protein expression resulting from withdrawal of leukaemia inhibitory factor (LIF), a cytokine required to maintain self-renewal in these cells. After iTRAQ labelling, we acquired MS/MS data at a depth of 20 DEEP SEQ fractions (Methods) on a 5600 Triple TOF mass spectrometer ( Fig. 2a ). A single experiment that required approximately 1 day for sample preparation and another 8 days for data acquisition yielded nearly 2 million MS/MS spectra and 0.6 million peptide spectral matches (PSMs) based on a search against the UniProt database that is composed of Swiss-Prot (16,502 mouse genes) plus Trembl (9,769 mouse genes) and contains 26,271 mouse genes in total. These PSMs corresponded to 180,867 peptides (≤1% false discovery rate (FDR), including chemical modifications). Following the convention described by Qeli et al . [17] , we mapped the set of 128,513 non-redundant peptide sequences into the genome as follows: first, 107,722 peptides were uniquely assignable to 9,818 gene IDs; we refer to these as ‘Class I’ peptides and genes, respectively ( Fig. 2b ). Of the remaining 20,791 peptides, 2,819 sequences mapped to at least two of another 1,737 gene IDs (‘Class II’ peptides and genes, respectively, Supplementary Data 2 ); importantly, Class II peptides do not map to Class I genes. The remaining 17,972 peptides (‘Class III’ peptides) map to multiple genes, including one or more Class I genes. Class III peptides are included in the count of total peptide detections but are not otherwise considered for purposes of protein identification. Cumulatively across three biological replicate experiments, comprising 24 days of data acquisition, we obtained ~5.9 million MS/MS spectra, ~1.8 million PSMs, and identified 211,535 non-redundant peptide sequences (178,167 Class I, 3,496 Class II and 29,872 Class III peptides, respectively). This peptide set encompassed 13,075 and 2,824 Class I and II genes, respectively ( Fig. 2c ), with the former (Class I genes) spanning 50% of UniProt and nearly 70% of the manually curated, non-redundant Swiss-Prot mouse database ( Fig. 2d ). 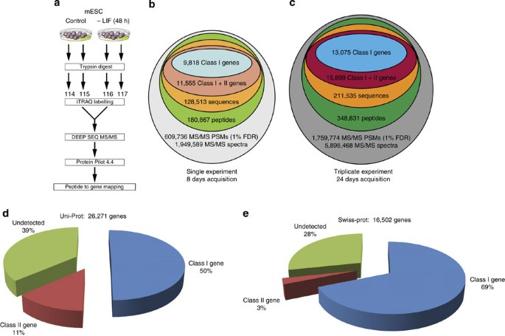Figure 2: DEEP SEQ mass spectrometry data spans 70% of protein-coding genes in mESCs. (a) mESC were cultured in the absence of LIF for 48 h. Proteins were solubilized and processed directly (for example, no sub-cellular or protein-level fractionation) for iTRAQ labelling (two replicates per condition), followed by DEEP SEQ mass spectrometry analysis. (b) A single, 20-fraction DEEP SEQ mass spectrometry analysis provided nearly 2 million MS/MS spectra, ~610,000 PSMs (<1% FDR) and 180,867 peptides corresponding to 128,513 unique peptide sequences. High-confidence (<1% FDR) peptide sequences were classified based on whether they mapped uniquely to mouse gene IDs (Class I peptide, Class I gene) or were shared across two or more mouse genes outside the set of Class I genes (Class II peptides, Class II genes). These data required 8 days of continuous acquisition time and yielded 9,818 Class I gene IDs. (blue). (c) Across biological triplicates, DEEP SEQ mass spectrometry analysis identified 13,075 Class I genes derived from ~5.9 million MS/MS spectra acquired over 24 days. These data spanned (d) 50% of all protein-coding genes in the UniProt database (26,271 entries). (e) The set of Class I peptides mapped unambiguously to nearly 70% of protein-coding genes in the manually annotated, non-redundant Swiss-Prot database (11,352 out of 16,502 total entries). Figure 2: DEEP SEQ mass spectrometry data spans 70% of protein-coding genes in mESCs. ( a ) mESC were cultured in the absence of LIF for 48 h. Proteins were solubilized and processed directly (for example, no sub-cellular or protein-level fractionation) for iTRAQ labelling (two replicates per condition), followed by DEEP SEQ mass spectrometry analysis. ( b ) A single, 20-fraction DEEP SEQ mass spectrometry analysis provided nearly 2 million MS/MS spectra, ~610,000 PSMs (<1% FDR) and 180,867 peptides corresponding to 128,513 unique peptide sequences. High-confidence (<1% FDR) peptide sequences were classified based on whether they mapped uniquely to mouse gene IDs (Class I peptide, Class I gene) or were shared across two or more mouse genes outside the set of Class I genes (Class II peptides, Class II genes). These data required 8 days of continuous acquisition time and yielded 9,818 Class I gene IDs. (blue). ( c ) Across biological triplicates, DEEP SEQ mass spectrometry analysis identified 13,075 Class I genes derived from ~5.9 million MS/MS spectra acquired over 24 days. These data spanned ( d ) 50% of all protein-coding genes in the UniProt database (26,271 entries). ( e ) The set of Class I peptides mapped unambiguously to nearly 70% of protein-coding genes in the manually annotated, non-redundant Swiss-Prot database (11,352 out of 16,502 total entries). Full size image Two recent reports [18] , [19] that sought to analyse global protein expression in mESC utilized pre-fractionation of sub-cellular compartments, proteins or peptides (or some combination) before LC-MS/MS. We took the union of published data from these studies and found that results from our DEEP SEQ platform encompass ~73% and ≥95% of the reported peptide and gene IDs, respectively, while adding a significant quantity of new sequence information ( Fig. 3a and Supplementary Data 3 ). Although the fractionation approaches, mass spectrometry instrumentation and database search engines varied across these three studies, we observed very similar physicochemical properties for peptides identified in each data set ( Fig. 3b ). To explore the dynamic range of proteins identified across these data, we next overlaid Class I and II genes derived from each peptide set with mRNA expression data for mESC [20] ( Fig. 3d and Supplementary Data 4 ). Class I genes identified in our data spanned the full dynamic range of gene expression, with new Class I peptides identified through additional replicate experiments generally mapping to genes expressed at lower levels. Moreover, peptides identified by the two previous studies [18] , [19] were biased to high-expression genes as compared with those in our data. Strikingly, the addition of Class II genes from our DEEP SEQ analysis improved overall proteome coverage only incrementally as compared with the set of Class I genes alone, with a small bias towards low-expression genes. Given the limitations of microarray data as a surrogate for protein expression, we next sought to compare our proteomic data with that from ribosomal profiling by RNA-seq, a technique that monitors protein translation on a genome-wide scale [21] . In a recent ribosomal profiling study, Ingolia et al . [9] measured translation of 12,674 transcripts from 19,022 protein-coding genes in mESC. Our set of Class I and II genes spanned an equivalent fraction of the total gene space (63%) and encompassed 81% of all translation events represented in the ribosomal profiling data ( Fig. 3e and Supplementary Data 5 ). Again, we observed that our deep-sequencing data spanned the entire dynamic range of protein translation as represented by ribosomal profiling, including significant coverage (~42%) of low-frequency translation events ( Fig. 3f ). As was observed in the comparison with gene expression by microarray, our data exhibited significantly higher coverage of low-expression genes as compared with that from previous studies of the mESC proteome [18] , [19] , while inclusion of DEEP SEQ Class II genes provided only a negligible improvement in proteome coverage. The latter observation is particularly notable, given that Class II genes are defined by shared peptides; as a result, the data for these gene products are ambiguous with respect to identification and quantification. For these reasons, we focused the remainder of our analyses exclusively on Class I genes. Collectively, these results suggest that our protein deep-sequencing platform provides accurate quantitative data for multiplexed stable isotope reagents while simultaneously maximizing the discovery potential in the analysis of complex mammalian proteomes. In fact, using very stringent criteria for unambiguous protein identification (Class I peptides), our DEEP SEQ mass spectrometry approach provides data that span the full dynamic range of mammalian protein expression. 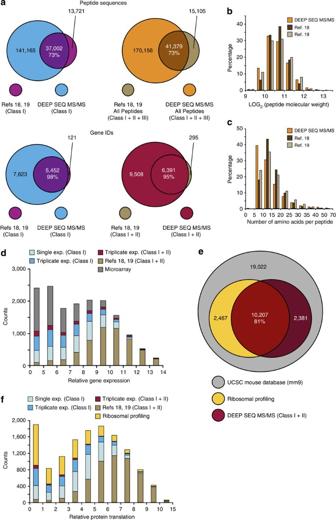Figure 3: Protein identification across the full dynamic range of gene expression and protein translation in mESC. (a) High-confidence peptides based on the union of published data from two previous mESC proteomic studies18,19were mapped to Class I and II gene IDs as described (see Methods) and compared with data from this study. High-confidence peptides identified in all three studies exhibited similar physicochemical properties, including (b) molecular weight distribution and (c) number of amino acids per peptide. Comparison of (d) Class I and II gene IDs with normalized mRNA levels in mESC demonstrates that DEEP SEQ mass spectrometry data spans the full range of gene expression. (e) The fraction of genes represented in the UCSC mouse database (grey) captured by ribosomal profiling (yellow) and DEEP SEQ mass spectrometry (red). The set of Class I and II genes identified herein encompassed 81% of protein translation events as represented by RNA-seq ribosomal profiling. (f) Overlay of ribosomal profiling data with that from DEEP SEQ mass spectrometry analysis demonstrates that the set of Class I genes spans the full dynamic range of protein translation in mESC. Figure 3: Protein identification across the full dynamic range of gene expression and protein translation in mESC. ( a ) High-confidence peptides based on the union of published data from two previous mESC proteomic studies [18] , [19] were mapped to Class I and II gene IDs as described (see Methods) and compared with data from this study. High-confidence peptides identified in all three studies exhibited similar physicochemical properties, including ( b ) molecular weight distribution and ( c ) number of amino acids per peptide. Comparison of ( d ) Class I and II gene IDs with normalized mRNA levels in mESC demonstrates that DEEP SEQ mass spectrometry data spans the full range of gene expression. ( e ) The fraction of genes represented in the UCSC mouse database (grey) captured by ribosomal profiling (yellow) and DEEP SEQ mass spectrometry (red). The set of Class I and II genes identified herein encompassed 81% of protein translation events as represented by RNA-seq ribosomal profiling. ( f ) Overlay of ribosomal profiling data with that from DEEP SEQ mass spectrometry analysis demonstrates that the set of Class I genes spans the full dynamic range of protein translation in mESC. Full size image Functional proteome coverage by DEEP SEQ mass spectrometry Regulatory proteins such as transcription factors, kinases and other signal transduction factors are often underrepresented in mass spectrometry-based whole-proteome studies. Hence, we next sought to evaluate the coverage of functional protein classes provided by our DEEP SEQ platform. We found that the set of Class I peptides mapped unambiguously to ≥40% of genes across gene ontology (GO) functional categories, regardless of the evidence filter used ( Fig. 4a ). We also observed that the coverage varied across categories, from nearly 100% for genes encoding ribosome and proteasome proteins to approximately 20% for transmembrane receptors; the same trend was observed for data derived from ribosomal profiling, suggestive of a general correlation between coverage and protein abundance. This hypothesis was further corroborated by mapping functional protein classes to gene expression in mESC ( Fig. 4c ). Consistent with these data, we found that replicate experiments tended to augment representation of proteins encoded by genes expressed at low levels. Overall, our set of stringently defined Class I genes spanned 52% of the functional proteome, on par with coverage provided by ribosomal profiling (56% coverage); importantly, our DEEP SEQ mass spectrometry data captured ≥70% of key regulatory protein classes, including kinases, phosphatases and transcription factors. 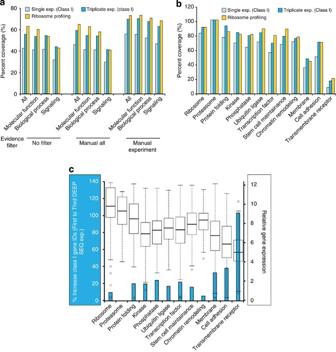Figure 4: DEEP SEQ mass spectrometry provides extensive coverage of the mammalian functional proteome. (a) Relative coverage provided by DEEP SEQ mass spectrometry and ribosomal profiling as a function of GO category and evidence filter. As defined by GO, ‘Manual All’ contains all curator-reviewed experimental and computational annotations, whereas ‘Manual Experiment’ includes only curator-reviewed annotations inferred from direct assay (IDA), physical interaction (IPI), mutant phenotype (IMP), genetic interaction (IGI), and expression pattern (IEP) evidence categories. (b) Relative coverage of GO protein families for DEEP SEQ mass spectrometry and ribosomal profiling analyses. Protein membership in each family is derived from the annotations within ‘Manual Experiment.’ (c) Relative mRNA expression level plotted in box-plot format (black and white,yaxis, right) as a function of GO protein families. Boxes encompass the interquartile range with respective median values indicated with stripes; whiskers represent 1.5 × the interquartile range with outliers shown as open circles. (blue,yaxis, left) Relative increase in GO protein family representation across bio-triplicate DEEP SEQ mass spectrometry analyses for Class I genes. Figure 4: DEEP SEQ mass spectrometry provides extensive coverage of the mammalian functional proteome. ( a ) Relative coverage provided by DEEP SEQ mass spectrometry and ribosomal profiling as a function of GO category and evidence filter. As defined by GO, ‘Manual All’ contains all curator-reviewed experimental and computational annotations, whereas ‘Manual Experiment’ includes only curator-reviewed annotations inferred from direct assay (IDA), physical interaction (IPI), mutant phenotype (IMP), genetic interaction (IGI), and expression pattern (IEP) evidence categories. ( b ) Relative coverage of GO protein families for DEEP SEQ mass spectrometry and ribosomal profiling analyses. Protein membership in each family is derived from the annotations within ‘Manual Experiment.’ ( c ) Relative mRNA expression level plotted in box-plot format (black and white, y axis, right) as a function of GO protein families. Boxes encompass the interquartile range with respective median values indicated with stripes; whiskers represent 1.5 × the interquartile range with outliers shown as open circles. (blue, y axis, left) Relative increase in GO protein family representation across bio-triplicate DEEP SEQ mass spectrometry analyses for Class I genes. Full size image Quantification of LIF-dependent functional proteome in mESC To explore the functional proteome characteristic of mESC, we next compiled two reference sets of pluripotent factors derived from genetic depletion screens [22] , [23] and proteins biochemically associated with the master regulatory transcription factors Oct4 and Nanog [24] , [25] , [26] ( Supplementary Data 6 ). The set of Class I genes from our biological triplicate analysis encompassed ~81% ( Fig. 5a ) and ~90% ( Fig. 5b ) of these reference gene sets, respectively, suggesting that our DEEP SEQ mass spectrometry platform can capture regulatory events associated with key mediators of pluripotency in mESC. A plot of quantitative data ( Fig. 5c ) revealed numerous proteins ( Table 1 ) whose expression level reproducibly increased or decreased in response to LIF withdrawal ( Supplementary Data 7 ). Query of these proteins against the functional and biochemical reference sets demonstrated an enrichment (Fisher’s exact test, P- value=2.1 E-5) for pluripotent factors ( Fig. 5d ). Biochemical validation ( Fig. 5e ) of LIF-mediated expression for a sub-set of proteins confirms the power of DEEP SEQ mass spectrometry to provide accurate quantification for multiplexed isobaric labels in the context of genome-wide proteome profiling. 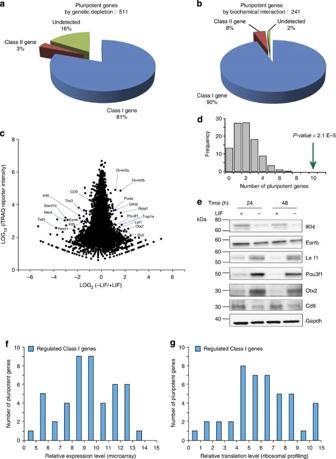Figure 5: DEEP SEQ mass spectrometry provides genome-wide proteome quantification in mESC subject to LIF withdrawal. The set of Class I gene IDs from bio-triplicate, 20-fraction DEEP SEQ mass spectrometry experiments encompassed (a) ~80% of murine pluripotent factors as defined by systematic genetic depletion assays22,23and (b) ~90% of the Nanog and Oct4 transcription factor network as defined through analysis of biochemical interactions24,25,26. (c) Scatter plot of iTRAQ log intensity versus log ratio for 13,075 class I gene IDs identified across bio-triplicate, 20-fraction DEEP SEQ mass spectrometry experiments. Individual iTRAQ signals for each high-confidence Class I peptide were summed across technical and biological replicates; these aggregate ratios were then combined to provide protein-level ratios. (d) Fisher’s exact test confirms that the set of regulated proteins (Table 1) identified by DEEP SEQ mass spectrometry analysis is enriched (two-sidedP-value=2 E-5) for pluripotent factors as defined by systematic loss-of-function and biochemical interaction assays. (e) Selected pluripotent and developmental factors were probed by western blot in mESC at 24 and 48 h after withdrawal of LIF. Left-most column indicates molecular weight markers. Overlay of regulated Class I gene products as detected by DEEP SEQ mass spectrometry with (f) relative gene expression as measured by microarray and (g) relative protein translation as measured by RNA-seq ribosomal profiling. Figure 5: DEEP SEQ mass spectrometry provides genome-wide proteome quantification in mESC subject to LIF withdrawal. The set of Class I gene IDs from bio-triplicate, 20-fraction DEEP SEQ mass spectrometry experiments encompassed ( a ) ~80% of murine pluripotent factors as defined by systematic genetic depletion assays [22] , [23] and ( b ) ~90% of the Nanog and Oct4 transcription factor network as defined through analysis of biochemical interactions [24] , [25] , [26] . ( c ) Scatter plot of iTRAQ log intensity versus log ratio for 13,075 class I gene IDs identified across bio-triplicate, 20-fraction DEEP SEQ mass spectrometry experiments. Individual iTRAQ signals for each high-confidence Class I peptide were summed across technical and biological replicates; these aggregate ratios were then combined to provide protein-level ratios. ( d ) Fisher’s exact test confirms that the set of regulated proteins ( Table 1 ) identified by DEEP SEQ mass spectrometry analysis is enriched (two-sided P- value=2 E-5) for pluripotent factors as defined by systematic loss-of-function and biochemical interaction assays. ( e ) Selected pluripotent and developmental factors were probed by western blot in mESC at 24 and 48 h after withdrawal of LIF. Left-most column indicates molecular weight markers. Overlay of regulated Class I gene products as detected by DEEP SEQ mass spectrometry with ( f ) relative gene expression as measured by microarray and ( g ) relative protein translation as measured by RNA-seq ribosomal profiling. Full size image Table 1 mESC protein expression (−LIF, 48 h). Full size table Continued advances in our understanding of genome variation [2] , gene expression [27] , [28] and translation [9] , driven in part by the advent of next-generation DNA/RNA-sequencing technologies [3] , have effectively re-kindled interest in experiments designed to maximize discovery potential and simultaneously quantify known genomic or other biomolecular events. Establishing a parallel trajectory for this paradigm in proteomics is complicated by the broad range of protein abundance, diverse repertoire and stoichiometry of post-translational modifications, as well as the stochastic nature of discovery-driven or shotgun MS/MS acquisition methods. In fact today, nearly two decades after Wilkins et al . [29] first coined the term ‘proteome’, the dynamic range of protein expression in mammalian systems has represented an insurmountable hurdle for genome-wide proteome quantification. Despite these obstacles, the functional content of protein-level data represents an important complement to genome-based studies, and hence there remains significant motivation to develop scalable platforms for proteomic analyses. To achieve true, genome-scale sequence coverage along with high-fidelity protein quantification, we sought to significantly improve the analytical figures of merit for each component of our DEEP SEQ mass spectrometry platform. First, the use of physicochemically orthogonal high-pH RP and SAX separation stages [16] , [30] coupled with a narrow-bore (25 μm i.d. ), extended-length (100 cm) low-pH analytical column [31] provides extreme temporal separation of peptides with an empirical peak capacity of ~1.3 E4. Our experience with online multidimensional separations [16] , [30] indicates that further optimization of first- and second-dimension eluent concentrations can yield an improved distribution of peptides across each separation dimension, ultimately providing deeper proteome coverage beyond the ~70% achieved herein. Second, the final dimension column geometry maintains the integrity of chromatographic separation at ultra-low effluent flow rates (~5 nl min −1 ), thus maximizing electrospray ionization efficiency [32] , [33] . Third, all separation stages in the DEEP SEQ configuration are implemented in microcapillary format and coupled in series, with the final dimension interfaced directly to the mass spectrometer, providing for fully automated operation, along with efficient capture and transfer of peptides across all separation stages. Based on a stringent peptide-to-gene ID criterion, our DEEP SEQ mass spectrometry analysis of mESC provided quantitative expression data for 11,352 out of 16,502 genes in Swiss-Prot (~69%, Fig. 2e ), a depth of coverage equivalent to a recent study in which RNA-seq ribosomal profiling was used to measure translation of 12,674 out of 19,022 (~66%) protein-coding genes contained in the UCSC mouse database [9] . Importantly, our data provide significant coverage (~70–85%) for key regulatory protein families, including kinases, ubiquitin ligases and transcription factors ( Fig. 4b ). In fact, proteins quantified on our deep-sequencing platform span the full dynamic range of corresponding gene expression and protein translation profiles ( Fig. 3d–f ). Not surprisingly, improvements in proteome coverage across triplicate experiments were most pronounced for low-expression protein families ( Fig. 4c ). The absence of protein-amplification strategies analogous to PCR, combined with the limited improvements in dynamic range offered by each generation of mass spectrometry hardware, places a disproportionate burden on separation techniques to achieve robust detection of low-abundance proteins. Despite numerous methodological studies, the choice of separation strategies that will provide the best combination of sample yield, experiment time and, ultimately, proteome coverage is unresolved. Our results refute the notion that analysis of tryptic peptides alone is insufficient to characterize proteins across a wide dynamic range of abundance. In practice, DEEP SEQ mass spectrometry achieves significantly higher proteome coverage ( Fig. 3a ) from only a fraction (<5%) of the input required by techniques that rely on protein- or cellular-level pre-fractionation [18] , [19] . In fact, although chromatographic and sub-cellular fractionation are slow and low-throughput compared with chemical amplification, the time required for our DEEP SEQ analysis (25 days for biological triplicates, including sample preparation) is not dramatically different from other recent attempts at protein deep sequencing by mass spectrometry (for example, 21 days for a study that relied on the use of protein-level fractionation and multiple enzymes [34] ), or for that matter genome-wide RNA-seq ribosomal profiling (9–12 days as described in a recent reveiw [35] ). Finally, it is worth noting that our DEEP SEQ approach provides the serendipitous benefit of a robust and streamlined sample-preparation protocol. Simple detergent solubilization, single-enzyme digestion, peptide desalting and iTRAQ labelling are somewhat reminiscent of the commoditized kits used in conjunction with next-generation DNA/RNA sequencing. The quality of peptide fractionation provided by our protein deep-sequencing platform is also evident in the analysis of a mixed-species iTRAQ quantification model ( Fig. 1a ). Even with contaminant species present in >30-fold excess relative to the target peptides, our DEEP SEQ mass spectrometry platform provided sufficient separation peak capacity to yield accurate iTRAQ ratios ( Fig. 1e ). These data are important in light of discrepancies reported between the throughput advantages afforded by multiplexed reagents and the well-documented limitations encountered when using these labels to quantify proteins in complex mixtures [11] , [12] , [13] , [36] . In fact, results from three of these studies [12] , [13] , [36] demonstrated unequivocally that two dimensions of peptide fractionation are insufficient to abrogate suppression of multiplexed ratios for analysis of samples intended to represent complex proteomes. Importantly, DEEP SEQ mass spectrometry provides a platform to reconcile these juxtaposed observations and fully leverage the advantages of isobaric reagents in studies designed to quantify proteome response to perturbation on a genome-wide scale. Moreover, recent reports [37] , [38] suggest the possibility of significant increases in the degree of multiplexing for these stable isotope reagents. These advances, along with improvements in mass spectrometry instrumentation [39] , [40] in addition to new chromatographic [41] , [42] , [43] and electrophoretic [44] , [45] , [46] separation platforms, will yield a concomitant increase in the throughput of DEEP SEQ mass spectrometry analysis. Finally, our data provide insight into the transition of mESC from a naive ground state, similar to that observed in the embryo inner cell mass before implantation, to a post-implantation epiblast-like stage (mouse epiblast stem cell) that is poised for directed differentiation [47] . LIF is a critical cytokine that supports self-renewal in mESC through the Jak-Stat and Pi3k-Akt signalling axes, while the opposing pathways, including Wnt-Gsk3β and Mek-Erk, mediate transcription programs that degrade pluripotent potential [48] . How these and other exogenous stimuli coordinately influence the core pluripotent genes (Oct4 and Sox2) and other peripheral factors to enforce the transcriptional ground state or mediate lineage commitment is not yet fully resolved. Strikingly, we detect regulated protein expression for downstream targets linked to each of these discrete pathways (Klf4, Klf5 (ref. 49 ), Lef1 (ref. 50 ), Esrrb, Tcfcp2l1 (ref 51 ) and Tbx3 (ref. 48 )). Proteins having roles in other developmental contexts (Otx2 (ref. 52 ), Pou3f1/Oct6 (ref. 53 ) and CD9 (refs 54 , 55 ), along with epigenetic factors (Dnmt3a/b) that are critical for high-fidelity gene expression [56] , were also regulated in a LIF-dependent manner. In addition to these studies that targeted specific genes or pathways, our DEEP SEQ analysis also quantified the majority of pluripotent factors previously defined by high-throughput functional genetic [22] , [23] and biochemical interaction [24] , [25] , [26] assays ( Fig. 5a ). Indeed, we reproducibly observed regulated expression for 50 proteins ( Table 1 ) and found that these were enriched for pluripotent and developmental genes ( Fig. 5d ). Importantly, this set of putative LIF-dependent protein targets spans the full dynamic range of gene expression and protein translation in mESC ( Fig. 5f ). Thus, though results presented herein represent a single time point in the LIF-mediated transition between naive and primed epiblast states, the depth and scale of these data provide compelling evidence that our DEEP SEQ mass spectrometry platform can capture the vast majority of the mESC functional proteome in the context of more complex experiments [57] , [58] designed to decipher individual contributions of the above pathways to self-renewal and lineage commitment. More generally, our DEEP SEQ mass spectrometry platform represents a powerful and scalable approach for genome-wide profiling of protein expression and post-translational modification status in mammalian systems. Cell culture Yeast cells were grown and processed under conditions similar to those described previously [30] . Saccharomyces cerevisiae , strain S288C, BY4741 (ATCC 201388, MATa his3Δ1 leu2Δ0met15Δ0 ura3Δ0) was grown in yeast extract peptone dextrose liquid medium to log phase, OD600 ≈0.7 at 30 °C. Cells were lysed by the addition of boiling SDS (50 mM Tris–HCl, pH 7.5, 7.5% SDS, 5% glycerol, 50 mM dithiothreitol (DTT) and 5 mM EDTA), followed by centrifugation, with the supernatant stored at −80 o C. Mouse embryonic stem cell (mESC) line J1 was generously provided by Dr Stuart Orkin (Dana-Farber Cancer Institute and Children’s Hospital, Boston, MA). Initially, 10 cm Nunclon tissue culture dishes (Thermo Fisher Scientific, Waltham, MA) were coated with 0.1% gelatin (EMD Millipore, Billerica, MA) at room temperature for 30 min. Gelatin was aspirated and J1 mESC were plated at a density of ~6 × 10 4 cm −2 in DMEM with high glucose supplemented with L -glutamine (Gibco Life Technologies, Carlsbad, CA), 15% embryonic stem cells validated FCS (Stem Cell Technologies, Vancouver, BC, Canada), 2-mercaptoethanol, nucleosides (EMD Millipore), nonessential amino acids (Gibco Life Technologies) and 10 ng ml −1 murine LIF6 (EMD Millipore). Perturbation experiments were performed by establishing J1 mESC under the above conditions and then removing LIF6 for 48 h. At the time of collection, plates were washed with cold PBS to remove serum proteins, and adherent cells were lysed by the addition of a boiling SDS (50 mM Tris–HCl, pH 7.5, 7.5% SDS, 5% glycerol, 50 mM DTT and 5 mM EDTA). Lysed cells were centrifuged, and the supernatant extract was stored at −80 o C. Sample preparation for DEEP SEQ analysis Proteins were precipitated by adding six volumes of cold (−20 °C) acetone and resolubilized in digestion buffer containing 8 M urea and 0.1 M NH 4 HCO 3 . Total protein levels were measured by BCA. DTT was added to a final concentration of 10 mM and incubated for 30 min at 60 °C, followed by addition of methyl methanethiosulfonate (MMTS) (Thermo Fisher Scientific) to 20 mM. After 30 min incubation in the dark at room temperature, excess MMTS was quenched by addition of DTT to a final concentration of 20 mM. Reduced and alkylated proteins were diluted in 0.1 M ammonium bicarbonate, followed by addition of trypsin, with overnight digestion at 37 °C and end-over-end rotation. Digested sample solutions were loaded onto SepPak C18 reverse phase cartridges (Waters Corp., Milford, MA) to remove urea and other salts. Eluted peptides (45% acetonitrile in water with 0.1% trifluoroacetic acid) were lyophilized by vacuum centrifugation. Peptides were labelled with 4-plex iTRAQ reagents (AB Sciex, Framingham, MA). Two aliquots of 0.2 μg yeast peptides were labelled with iTRAQ 114 and 115. Separately, two other aliquots of 1.0 μg yeast peptides were labelled with iTRAQ 116 and 117. In addition, two aliquots of 6.3 μg peptides from mESC were labelled with iTRAQ 114 and 116. For the mESC perturbation experiment, peptides from the cells incubated without LIF were labelled as technical replicates with iTRAQ 116 and 117, whereas peptides from the cells incubated with LIF were labelled as technical replicates with iTRAQ 114 and 115. For each reaction, peptides were resuspended in 500 mM triethylammonium bicarbonate and mixed with the appropriate iTRAQ reagent in ethanol. Labelling was allowed to proceed at room temperature for 1 h, and samples were then combined and dried by vacuum centrifugation. Fresh aliquots of mESC were processed as described above to provide biological triplicates. DEEP SEQ multi-dimension separation Three-dimension peptide separation was performed on a modified Waters Corp. NanoAcquity UHPLC system with binary and isocratic pumps, along with an autosampler and additional 6-port, 2-position valve (Valco, Austin, TX). The first-dimension RP column consisted of a 200-μm i.d. capillary packed with 20 cm of 5 μm diametre (dia.) XBridge C18 resin (Waters Corp.). An anion-exchange column (200 μm i.d. × 20 cm) was packed with 5 μm dia. SAX resin (Sepax Technologies, Neward, DE) and connected to the outlet of the first-dimension RP column. The third dimension consisted of RP pre- (100 μm i.d. × 4 cm of 10 μm dia. POROS 10R2 resin) and analytical (25 μm i.d. × 100 cm of 5 μm dia. Monitor C18 Column Engineering, Ontario, CA), with integrated 1 μm dia. emitter tip columns configured in a vented geometry [59] , [60] . The autosampler picked up and delivered either peptide samples or first (acetonitrile in 20 mM ammonium formate, pH 10) and second (KCl in 20 mM ammonium formate, pH 10) dimension eluents at 2 μl min −1 through the sample loop. Injection of each first- or second-dimension eluent constitutes a ‘DEEP SEQ fraction’ ( Supplementary Data 8 ). The binary pump delivered 0.1% formic acid at 8 μl min −1 to dilute the organic content and acidify the first/second-dimension effluent before the third-dimension pre-column, or provided for gradient elution (2–50% B in 580 min, A=0.1% formic acid, B=acetonitrile with 0.1% formic acid) of peptides from the third-dimension RP columns for LC-MS/MS analysis at a flow rate of ~5 nl min −1 . A Digital PicoView electrospray source platform (New Objective, Woburn, MA) was used on both the Orbitrap XL and 5600 Triple TOF mass spectrometers to automatically position the emitter tip at the source inlet during LC-MS/MS acquisition or beneath a gravity-driven drip station during injection of peptide samples or first/second-dimension eluents. DEEP SEQ sample capacity and experiment time Based on our published and unpublished studies, we estimate that the total loading capacity of our first-dimension RP column (200 μm i.d. × 20 cm) is currently ~100 μg. The DEEP SEQ platform is easily tailored to a variety of sample types. Generally, first- and second-dimension eluent concentrations in a range of 7–55% acetonitrile and 10–300 mM KCl represent the useful boundaries for peptide elution. Importantly, our experience to date suggests that these conditions are robust with respect to biological input, obviating the need to run repeated pilot experiments for every sample. Total time of analysis is another important consideration when using multidimensional fractionation techniques. For example, DEEP SEQ experiments performed at a depth of 20 fractions required 8 days for data acquisition. System reliability is particularly important, given that a single, DEEP SEQ mass spectrometry analysis will typically require several days of continuous instrument time. Importantly, all data presented herein were acquired using a single 25-μm i.d. × 100-cm resolving column, demonstrating the robustness of our platform. DEEP SEQ mass spectrometry data-acquisition parameters The LTQ-Orbitrap XL mass spectrometer (Thermo Fisher Scientific) was operated in data-dependent mode, such that the top 10 most abundant precursors in each MS scan were subjected to MS/MS in both collisionally activated dissociation (CAD) and higher energy collisional dissociation (HCD) mode (CAD in the linear trap, normalized collision energy=35%, precursor isolation width=1.9 Da, intensity threshold for precursor selection=20,000 HCD in the orbitrap, normalized collision energy=47%, precursor isolation width=1.0 Da and intensity threshold for precursor selection=20,000). Dynamic exclusion was enabled with a repeat count of 1 and exclusion duration set to 20 s. Electrospray voltage was 2.2 kV. We enabled the Lock Mass feature and selected m/z =445.120025 ([Si(CH 3 ) 2 O] 6 ) as the internal calibrant. The 5600 Triple TOF (AB Sciex) was operated in information-dependent mode, with the top 50 precursors (charge state +2 to +5, >100 counts) in each MS scan (800 ms, scan range 350–1,500 m/z ) subjected to MS/MS (minimum time 140 ms, scan range 100–1,400 m/z ). A dynamic exclusion window of 20 s was used with unit resolution for precursor isolation. Electrospray voltage was 2.2 kV. Native DEEP SEQ mass spectrometry data files along with Mascot generic format (MGF) peak lists are available for download at: http://blaispathways.dfci.harvard.edu/mz/?id=doi:10.1038/ncomms3171 . DEEP SEQ mass spectrometry data processing Our application programming interface (API) based multiplierz software framework was used to extract and format MS/MS data from the Orbitrap XL for subsequent search against the UniProt mouse database (downloaded on 02 November 2011) and a S. cerevisiae database (downloaded from http://www.yeastgenome.org/01/06/2010 ). MS/MS data were searched using Protein Pilot V4.4 (AB Sciex) with the following parameters: instrument=‘Orbi/FT MS (sub-p.p.m. ), LTQ MS/MS’ for data acquired with the Orbitrap XL or ‘5600 Triple TOF’ for data acquired with the 5600 Triple TOF mass spectrometer. A fixed modification of +42 corresponding to MMTS of cysteine was also included. The sample type was set to ‘iTRAQ 4-plex (peptides labelling)’. All PSMs from bio-triplicate acquisitions were combined for the FDR assessment. Only those peptides with scores at or above a PSM FDR threshold of 1% were further considered. All peptides were mapped back to the genome without consideration of splice isoforms from the same gene. Following the procedure of Qeli and Ahrens [17] , peptides passing the 1% FDR filter were classified as either ‘unique’ or ‘shared’ based on whether they could be assigned to only one or more than one gene, respectively. Class I genes were defined as those identified only by uniquely assignable peptides. Class II genes were identified based on shared peptides that could not be assigned to any Class I gene. The results reported herein are based on Class I and Class II genes; no Class III genes were included in our analyses. Multiplierz scripts were used to programmatically generate extracted ion chromatograms (XICs) and calculate corresponding peak widths for all identified peptides. To estimate the orthogonality of peptide fractionation, the number of unique peptides identified in each third-dimension LC-MS/MS run was represented as a circle of proportional diameter and projected onto a 2D plot at the corresponding first-dimension acetonitrile ( x axis) and second-dimension salt ( y axis) concentrations used in the experiment. Linear regression was performed using the function stats.linregress from Numpy version 1.4.1, with each unique peptide sequence used as a separate data point. In the mixed-species quantification experiments, the iTRAQ 116/iTRAQ 114 and iTRAQ 117/iTRAQ 115 ratios were first normalized based on all spectra identified (final normalization factor was 1.14). We used R scripts to create box plots for all iTRAQ ratios. For the quantitative analyses of mESC, we summed iTRAQ channels in each biological condition (±LIF) for Class I peptides to generate a final ratio for each Class I gene. Across three biological triplicate experiments, a protein was considered to be regulated in expression ( Table 1 ) if the following criteria were met in two out of the three experiments: (i) the iTRAQ intensities exceeded 200 counts and (ii) the Log 2 iTRAQ ratio was ≥1 or ≤−1. Enrichment of pluripotent factors within the set of genes whose expression was reproducibly regulated across bio-triplicate experiments was estimated using a Fisher’s exact test. A null distribution and two-sided P -value were calculated based on code freely available at: ( http://research.microsoft.com/en-us/um/redmond/projects/MSCompBio ). Comparisons with mESC microarray and ribosomal profiling data Comparison of DEEP SEQ mass spectrometry data with that from ribosome profiling for mESC was performed as follows: the UCSC mouse genome database (mm9) ( http://hgdownload.soe.ucsc.edu/goldenPath/mm9/database/ ) was downloaded on 02 October 2012. We aligned the peptides identified in triplicate DEEP SEQ mass spectrometry analyses against sequences in the UCSC database. A similar alignment was performed for mESC ribosomal profiling data previously reported [9] . In 1,034 cases, we were unable to reconcile gene names from the UCSC and UniProt databases; these genes were removed from further consideration. Average gene expression levels across three wild-type mESC lines (B21, J1 and R1) were calculated using published data sets (accession codes GSM338369, GSM338371 and GSM338373) (ref. 20 ). We used the R/Bioconductor software environment to re-normalize all microarray data based on the Robust Multi-array Average (RMA) method and to re-map all probe sequences to Entrez Gene IDs using a custom Chip Definition File from the Michigan Microarray Lab (version 13). The average mRNA expression level (in Log 2 space) between the three arrays was calculated, and the Entrez Gene IDs were converted to UniProt gene symbols. UniProt entries mapping to more than one Entrez Gene ID were excluded. The final list contained 15,705 entries of average Log 2 expression value/UniProt gene symbol pairs. GO and reference gene sets for pluripotency Positive reference sets of pluripotent genes were created from RNAi screening data downloaded from two previous studies [22] , [23] . Similarly, pluripotency reference genes based on biochemical interactors of Nanog and Pou5f1 (Oct4) were created from three previous studies [24] , [25] , [26] . The GO database was downloaded on 15 March 2012. The GO subcategories were filtered based on different identifiers: molecular function (GO:0003674), biological process (GO:0008150), signalling (GO:0023052), ribosome (GO:0005840), proteasome (GO:0000502), protein folding (GO:0006457), kinase (combination of GO:0004672 and GO:0016301), phosphatase (combination of GO:0016791 and GO:0004721), ubiquitin ligase (GO:0004842), transcription factor (combination of GO:0006351 and GO:0008134), stem cell maintenance (GO:0019827), chromatin remodelling (GO:0006338), membrane (GO:0016020), cell adhesion (GO:0007155) and transmembrane receptor (GO:0004888). Western blotting Protein lysates from ~3 × 10 5 murine ESC (about 30 μg total protein) incubated with or without LIF were separated on 4–12% Bis-Tris gels (Life Science) under reducing conditions and transferred onto polyvinylidene difluoride membranes. The blot was stained with antibodies against Lef1 (Cell Signaling Technology, 1:1,000), Pou3f1 (Abcam, 1:1,000), Esrrb (Cell Signaling Technology, 1:1,000), Otx2 (Abcam, 1:1,000), Klf4 (Cell Signaling Technology, 1:1,000), Cd9 (Abcam, 1:1,000) and Gapdh (Cell Signaling Technology, 1:6,000). The bands were visualized by enhanced chemiluminescence (SuperSignal West Femto Chemiluminescent Substrate; Thermo). How to cite this article: Zhou, F. et al . Genome-scale proteome quantification by DEEP SEQ mass spectrometry. Nat. Commun. 4:2171 doi: 10.1038/ncomms3171 (2013).